Orbital Asian summer monsoon dynamics revealed using an isotope-enabled global climate model The Asian summer monsoon dynamics at the orbital scale are a subject of considerable debate. The validity of Asian speleothem δ 18 O records as a proxy for summer monsoon intensity is questioned together with the ultimate forcing and timing of the monsoon. Here, using the results of a 150,000-year transient simulation including water isotopes, we demonstrate that Asian speleothem δ 18 O records are not a valid proxy for summer monsoon intensity only at the orbital timescale. Rather, our results show that these records reflect annual variations in hydrologic processes and circulation regime over a large part of the Indo-Asian region. Our results support the role of internal forcing, such as sea surface temperature in the equatorial Pacific, to modulate the timing of monsoon precipitation recorded in paleo-proxies inside the Asian region. The Asian summer monsoon is a major component of the climate system [1] and affects the economical prosperity of vast, heavily populated regions [2] . Characterization of past monsoons can improve our knowledge about monsoon dynamics and their future impacts. As paleoclimatic records are increasingly used to evaluate the ability of numerical climate models to correctly simulate the climate system, it is also critical to assess the proxies used to document monsoons. To date, the stable isotope signal (δ 18 O) archived in South Asian speleothems from Hulu [3] (32°30′N, 119°10′E), Sanbao [4] (31°40′N, 110°26′E) and Dongge [5] (25°170′N, 108°50′E) caves constitute among the best-dated records susceptible to deliver past hydrological information over the late Quaternary. These deposits have been widely interpreted as records of changing intensity of the summer monsoon precipitation at orbital scales. However, interpretation of the speleothem δ 18 O record is complex and is a subject of considerable debate [3] , [4] , [5] , [6] , [7] , [8] , [9] , [10] , [11] , [12] , [13] , [14] , [15] , [16] , [17] , [18] , [19] . Studies point to the potential control of seasonality, as well as large-scale atmospheric circulation effects in addition to the amount of Asian summer monsoonal rainfall on the δ 18 O signal [11] , [12] , [17] , [18] . The lack of consensus also reveals the deficits in our understanding of monsoon sensitivity to changes in the most basic boundary conditions. The speleothem δ 18 O records over Asia seem to be forced mainly and directly by local orbitally forced insolation [3] , [4] , [5] , [9] , [20] , [21] . On the contrary, a large variety of other Indo-Asian summer monsoonal records (marine and continental records documenting winds and precipitation) suggest a sensitivity to northern hemisphere summer sensible heating (insolation), the timing of energy release from the southern hemisphere Indian Ocean and the timing of global ice-volume minima [6] , [7] , [11] , [12] , [13] , [14] , [16] . In our study, we quantify the roles of these different driving factors on the dynamics of the Asian monsoon and explore the impact of seasonality by analysing numerical experiments performed with an isotope-enabled global climate model (Methods). A decisive advantage of isotope-enabled models is their ability to directly simulate measured quantities (in the present case, δ 18 O), so that the results can be directly compared with speleothem data. This enables us to assess the nature of the δ 18 O signal in South Asian speleothems, to establish whether they are a valid proxy for summer monsoon intensity and reveal the ultimate forcing of Asian monsoon precipitation at the orbital scale. Data-model comparison for south Asia annual calcite δ 18 O The transient simulation results for the δ 18 O in precipitation and atmospheric temperature averaged over the South Asian region (~17°N–33°N and 87°E–116°E), encompassing Sanbao, Hulu and Dongge cave locations, exhibit important variability over the last 150,000 years ( Figs 1 and 2 ). Large variations of the δ 18 O in precipitation (up to 4‰ in amplitude) occur and seem related to orbital changes (precession and obliquity) that drive northern hemisphere insolation and are a reference for monsoon proxies [11] ( Fig. 1a,e ). On the other hand, atmospheric temperature variations (up to 3 °C in amplitude) slightly lag northern hemisphere ice-volume changes ( Fig. 1b,c ). The modelled annual temperatures are regionally consistent with reconstructed variations between the last glacial maximum and present (~3 °C, Methods). 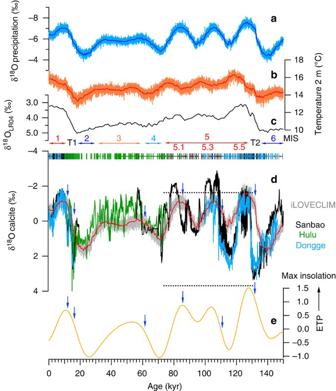Figure 1: Data–model comparison for calcite δ18O in South Asia. (a) Annual mean δ18O in precipitation in South Asia (~17°N–33°N and 87°E–116°E) withiLOVECLIM. (b) Same asabut for atmospheric temperature. (c) δ18O stack of benthic foraminifera (LR04) as a proxy for ice-volume changes46. MIS denote Marine Isotopic Stages and T1–T2 denote Termination 1 and 2, respectively. (d) Comparison between annual mean calcite δ18O computed withiLOVECLIM (Methods) and Sanbao, Hulu and Dongge cave records3,4,5(indicated with different colours). Data and model results are shown as deviations from their respective long-term means. Speleothems U/Th control points are indicated3,4,5. Blue arrows indicate periods of weak monsoon intervals (WMIs) at times of maximum northern hemisphere insolation9,24. The dashed line highlights the different amplitudes of monsoon maxima during MIS 5. A low-pass filter (200 years) has been applied to the records ina) (full blue line), (b) (full red line) and (d) (full red line) that correspond to the lower resolution in speleothems. (e) ETP is constructed by normalizing and stacking Eccentricity, Tilt (obliquity) and negative Precession47. The dashed line highlights the different amplitude of insolation maxima during MIS 5. Figure 1: Data–model comparison for calcite δ 18 O in South Asia. ( a ) Annual mean δ 18 O in precipitation in South Asia (~17°N–33°N and 87°E–116°E) with i LOVECLIM. ( b ) Same as a but for atmospheric temperature. ( c ) δ 18 O stack of benthic foraminifera (LR04) as a proxy for ice-volume changes [46] . MIS denote Marine Isotopic Stages and T1–T2 denote Termination 1 and 2, respectively. ( d ) Comparison between annual mean calcite δ 18 O computed with i LOVECLIM (Methods) and Sanbao, Hulu and Dongge cave records [3] , [4] , [5] (indicated with different colours). Data and model results are shown as deviations from their respective long-term means. Speleothems U/Th control points are indicated [3] , [4] , [5] . Blue arrows indicate periods of weak monsoon intervals (WMIs) at times of maximum northern hemisphere insolation [9] , [24] . The dashed line highlights the different amplitudes of monsoon maxima during MIS 5. A low-pass filter (200 years) has been applied to the records in a ) (full blue line), ( b ) (full red line) and ( d ) (full red line) that correspond to the lower resolution in speleothems. ( e ) ETP is constructed by normalizing and stacking Eccentricity, Tilt (obliquity) and negative Precession [47] . The dashed line highlights the different amplitude of insolation maxima during MIS 5. 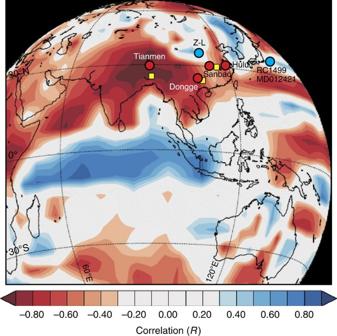Figure 2: Spatio-temporal correlation between δ18O in precipitation and precipitation rate withiniLOVECLIM. The spatio-temporal correlation was realized between δ18O in precipitation of the South Asian region (~17°N–33°N and 87°E–116°E) and grid cells precipitation rate. A 100-year moving average was applied prior to the correlation to obtain a mean climatology. Red dots indicate the location of speleothem records discussed in the study with a timing that lags the minimum of precession by ~3 kyr3,4,5,9,20,21. Blue dots indicate the location of monsoon precipitation records with a mean timing that lags the minimum of precession by ~8 kyr (refs11,48). Yellow squares indicate the location of Global Network of Isotopes in Precipitation (GNIP) stations49(Supplementary Fig. 5). Full size image Figure 2: Spatio-temporal correlation between δ 18 O in precipitation and precipitation rate within i LOVECLIM. The spatio-temporal correlation was realized between δ 18 O in precipitation of the South Asian region (~17°N–33°N and 87°E–116°E) and grid cells precipitation rate. A 100-year moving average was applied prior to the correlation to obtain a mean climatology. Red dots indicate the location of speleothem records discussed in the study with a timing that lags the minimum of precession by ~3 kyr [3] , [4] , [5] , [9] , [20] , [21] . Blue dots indicate the location of monsoon precipitation records with a mean timing that lags the minimum of precession by ~8 kyr (refs 11 , 48 ). Yellow squares indicate the location of Global Network of Isotopes in Precipitation (GNIP) stations [49] ( Supplementary Fig. 5 ). Full size image We computed annual mean calcite δ 18 O from simulated δ 18 O in precipitation and atmospheric temperature (Methods) and compared the results with speleothem calcite δ 18 O data ( Fig. 1d ). Considering a change of 0.26‰/°C [22] , the change in atmospheric temperature (maximum 3 °C) over the last 150,000 years can only account for a maximum of 0.8‰ of the calcite δ 18 O signal of speleothems. We therefore conclude that the mean annual calcite δ 18 O signal of South Asian speleothems is mainly controlled by δ 18 O in precipitation changes ( Fig. 1 ). To determine the sensitivity to remote changes on the δ 18 O in precipitation at cave sites, we calculated the spatio-temporal correlation of the South Asian signal with precipitation rate ( Fig. 2 ), atmospheric temperature and δ 18 O in surface seawater ( Supplementary Fig. 1 ) over the Indo-Asian region for the last 150,000 years. South Asian annual mean δ 18 O in precipitation correlates very well with rainfall over a large part of the Indo-Asian region, but not with atmospheric temperature ( Fig. 2 ; Supplementary Fig. 1 ). The correlation is stronger over India and the Arabian Sea than over South-East Asia, indicating that the signal is not entirely related to local precipitation amount. The observed correlations between δ 18 O in precipitation and δ 18 O in surface seawater in the tropical South Indian Ocean and Pacific Ocean highlights potential distinct source region for the δ 18 O in precipitation signal, as observed today [11] ( Supplementary Fig. 1 ). We can therefore conclude that the calcite δ 18 O signal of speleothems is a good proxy to document the annual variations of hydrologic processes and circulation regime over a large part of the Indo-Asian region. The spatial correlation reveals why the calcite δ 18 O signal is found to be very consistent between speleothem records ( Fig. 2 ; Supplementary Fig. 1 ). We realized simulations with orbital and ice-sheet forcing only to investigate their respective role on South Asian precipitations ( Supplementary Fig. 2 ). Ice-sheet changes and orbital changes both play an important role in driving the annual precipitation and calcite δ 18 O signals with a different timing. Phase analyses in the precession band (23,000 years), which is so far extremely debated [11] , reveal that the minimum calcite δ 18 O signal using ice-sheet forcing lags the minimum of precession (Pmin, June 21 perihelion) by ~4 kyr, whereas the calcite δ 18 O signal using orbital forcing only led Pmin by ~600 years ( Supplementary Fig. 3 ). Calcite δ 18 O of speleothem records lag Pmin by ~3 kyr [11] . The annual calcite δ 18 O signal simulated with i LOVECLIM (including all forcings) lag Pmin by ~1 kyr ( Supplementary Fig. 3 ). We can therefore conclude that the waxing and waning of northern hemisphere ice sheets exerts an influence on the timing of hydrologic processes in Asia as already suggested [23] . The remaining 2 kyr of difference that is observed between the simulated calcite δ 18 O signal and speleothem records could be attributed to the effect of weak monsoon intervals (WMIs) ( Supplementary Fig. 3 ). Indeed, the computed annual mean calcite δ 18 O signal is in good agreement with Asian speleothem data, but disagreements occur during periods corresponding to maximum insolation ( Fig. 1d,e ). These periods have been previously called WMIs in speleothem records [9] , [24] and are not reproduced in the model. The proposed explanation for such WMIs is the effect of ice-sheet collapses in the northern hemisphere together with inter-hemispheric interactions, which act to reduce monsoon strength [9] , [17] , [19] , [24] . As we have not included freshwater fluxes induced by ice-sheet collapses in our transient simulation, we cannot expect to reproduce such events. Our results therefore demonstrate that the orbital forcing, Greenhouse Gases (GHGs) and changes in ice-sheet size (that is, the forcings included in our simulation) are not sufficient processes to explain the WMIs. The absence of ice-sheet collapse events could also explain the difference in amplitude between the computed annual mean calcite δ 18 O and speleothem data during Marine Isotopic Stage (MIS) 3 ( Fig. 1d ; Supplementary Fig. 4 ). Another disagreement in terms of signal amplitude can be observed during MIS 5 ( Fig. 1d ; Supplementary Fig. 4 ). Speleothem data at Sanbao indicate higher negative values for monsoon maxima during MIS 5.3 and 5.1 compared with other Asian speleothem δ 18 O records at Tianmen and Dongge [20] , [21] . The modelled values are in accordance with Tianmen and Dongge data during MIS 5.1 and 5.3, with a difference of amplitude between MIS 5.3–5.1 and 5.5 linked to orbital and ice-sheet forcings ( Supplementary Fig. 2 ). We hypothesize that the differences observed at Sanbao could be linked to potential biases that occur in the natural environment, soil zone, epikarst and cave system in South Asia. Asian monsoon precipitation seasonality and forcing To investigate the seasonal contribution to the mean annual δ 18 O signal and assess the use of South Asian speleothem records as a summer monsoon proxy, we realized 30 years of daily simulation every 5,000 years over the last 150,000 years (Methods). In Asia, δ 18 O in precipitation and atmospheric temperature results for the present day satisfyingly agrees in term of qualitative seasonal changes when compared with Global Network of Isotopes in Precipitation (GNIP) station measurements ( Supplementary Fig. 5 ). Results over the past 150,000 years indicate that the summer monsoon rarely contributes more than half of the annual precipitation, as it is observed today [11] ( Fig. 3a ; Supplementary Fig. 5 ). Differences in the value for δ 18 O in calcite can also be observed between the modelled summer and annual signals over the past 150,000 years (up to 1.5‰) ( Fig. 3b ). In addition, influence of non-monsoonal variations on calcite δ 18 O signal of speleothems exists with a significant strength ( Supplementary Fig. 6 ). Furthermore, the calcite δ 18 O signal during the summer season is in phase with Pmin contrary to annual and non-monsoon calcite δ 18 O signals ( Supplementary Figs 3 and 7 ). This is probably because ice-sheet influence is important during the complete annual cycle and not only during the summer season. Therefore, the δ 18 O calcite signal of speleothems cannot be considered as a summer monsoonal proxy only, but rather as a proxy of the mean annual hydrological cycle for which seasonal contributions modulated the amplitude and timing of the recorded signal ( Fig. 3a,b ; Supplementary Fig. 7 ). 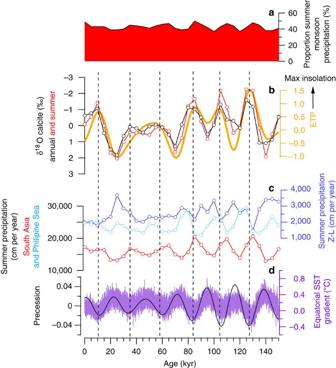Figure 3: Asian monsoon precipitation seasonality and forcing. (a) Proportion of summer monsoon precipitation in South Asia compared with total annual (~17°N–33°N and 87°E–116°E) withiLOVECLIM (Methods). (b) Comparison between annual and summer monsoon δ18O in calcite in South Asia (~17°N–33°N and 87°E–116°E) withiLOVECLIM. ETP that is constructed by normalizing and stacking Eccentricity, Tilt (obliquity) and negative Precession47is indicated. (c) Comparison between summer monsoon precipitation in South Asia (~17°N–33°N and 87°E–116°E) and in North-East Asia: Philipine Sea-NW Pacific (~33°N–39°N and 144°E–150°E) and Z-L Loess region (~33°N–39°N and 104°E–110°E). (d) Pacific cross-equatorial sea-surface temperature gradient between ~5–15°S and 5–15°N, averaged for 80°W–150°W. The precession index is indicated47. Dashed vertical lines indicate periods of minimum calcite δ18O in South Asia. Figure 3: Asian monsoon precipitation seasonality and forcing. ( a ) Proportion of summer monsoon precipitation in South Asia compared with total annual (~17°N–33°N and 87°E–116°E) with i LOVECLIM (Methods). ( b ) Comparison between annual and summer monsoon δ 18 O in calcite in South Asia (~17°N–33°N and 87°E–116°E) with i LOVECLIM. ETP that is constructed by normalizing and stacking Eccentricity, Tilt (obliquity) and negative Precession [47] is indicated. ( c ) Comparison between summer monsoon precipitation in South Asia (~17°N–33°N and 87°E–116°E) and in North-East Asia: Philipine Sea-NW Pacific (~33°N–39°N and 144°E–150°E) and Z-L Loess region (~33°N–39°N and 104°E–110°E). ( d ) Pacific cross-equatorial sea-surface temperature gradient between ~5–15°S and 5–15°N, averaged for 80°W–150°W. The precession index is indicated [47] . Dashed vertical lines indicate periods of minimum calcite δ 18 O in South Asia. Full size image On the basis of our modelling results, the dominant control on South Asia summer monsoon precipitation is the orbital forcing with a lead of ~2.5 kyr compared with Pmin ( Supplementary Fig. 7 ). A previous modelling study forced by orbital changes only observed a lead of ~1.5 kyr between summer precipitation in Asia and Pmin [25] ( Supplementary Fig. 7 ). An in-phase relationship is found between summer precipitation in Asia and Pmin in the CLIMBER-2 model that includes varying ice sheets and greenhouse gas concentrations [26] . This different result in comparison with i LOVECLIM may be attributed to the fact that CLIMBER-2 does not include all relevant atmospheric teleconnections to evaluate how exactly ice-sheet-related changes in the positions of the Westerlies and Siberian High affect the Asian monsoon [26] . Interestingly, summer δ 18 O in precipitation and calcite δ 18 O signals are phased with Pmin ( Supplementary Fig. 7 ; Supplementary Table 1 ). The lag in comparison with maximum summer precipitation could therefore reflect isotopic sources and circulation regime effects, again pointing to a complexity of the isotopic signal recorded in speleothems. The different timing observed between monsoonal precipitation paleoclimate-records in Asia ( Fig. 2 ) requires an explanation. We observe in our model an anti-phase in the response of annual mean precipitation between the South Asia and North-East Asia ( Fig. 2 ) that also exists for the summer monsoon precipitation ( Fig. 3c ; Supplementary Fig. 7 ; Supplementary Table 1 ). This pattern was observed in a global climate numerical model [15] forced by insolation alone and could be linked to different modes of tropical Pacific sea surface temperature (SST). We investigate Pacific tropical SST gradient in our model and find changes in-phase with the precession ( Fig. 3d ; Supplementary Table 1 ) as was also observed in some previous modelling studies [15] , [27] , [28] . This Pacific SST gradient significantly correlates with the anti-phased response of precipitation between the South Asia and North-East Asia contrary to the Indian SST gradient ( Fig. 2 ; Supplementary Fig. 8 ). The SST warming in the eastern tropical Pacific is associated with weaker trade winds ( Supplementary Fig. 8 ). This configuration can produce an anticyclonic anomaly over the northwestern Pacific and lead to an intensified East-Asian summer monsoon at times of precession maxima [15] . More water vapour from the tropical ocean is transported by stronger monsoon and shifts the rain belt to the northern East-Asian region, resulting in enhanced precipitation there and reduced precipitation in the south as observed in our simulation results ( Fig. 3 ; Supplementary Fig. 8 ). We conclude that ocean internal forcing in the climate system can lead to the different phases observed in precipitation palaeo-proxies within the Asian monsoon region ( Figs 2 and 3 ; Supplementary Fig. 8 ). Similarly, the monsoon winds could be affected by such ocean internal feedback not only from the Pacific [15] , but also from the southern Indian Ocean [6] , [7] , [11] , [12] , [13] , [14] , [16] , [29] and lead to different timing. Our study therefore highlights a complex Asian monsoon dynamic with distinct response inside the monsoon system. Transient simulation setup for i LOVECLIM We used the i LOVECLIM model, a derivative of the LOVECLIM model [30] because of its computing efficiency. Although our model experiences some weaknesses caused by its spatial resolution and simplified convective physics (in particular, the summer precipitation is underestimated and the low-level geopotential ridge over the North Pacific is shifted northward 10 degrees in latitude compared with observations), LOVECLIM was previously successfully applied in the Asian monsoon region for qualitative assessment of the connections between ice sheets and sub-tropical dynamics [31] and reconstruction of past monsoonal precipitation [32] , [33] . Nikolova et al . [34] conducted a detailed analysis of the climate of the last interglacial simulated by two climate models of different complexities, CCSM3 and LOVECLIM. In their study, JJA surface temperature anomalies compare well. Both CCSM3 and LOVECLIM simulate significantly stronger northern monsoons during MIS-5e, in good agreement with proxy-based reconstruction. The surface wind and moisture transport during MIS-5e are in good agreement with water vapour supply over east Asia coming mainly from the Indian Ocean and secondarily from the South China Sea and western Pacific Ocean. The simulated upper level (200 hPa) tropical easterly jet anomaly is stronger in both models during MIS-5e. LOVECLIM also compared well with other models for the simulation of monsoon precipitations: FAMOUS and HadCM3 snapshot simulations over the East-Asian region for the last 90,000 years [33] ( Supplementary Fig. 9 ). Details regarding the implementation and validation of water isotopes in i LOVECLIM can be found in Roche [35] , Roche and Caley [36] and Caley and Roche [37] . We used an accelerated forcing technique, where irradiance, GHGs and ice sheets are updated with an acceleration factor 10. Ice-sheet forcing is from Ganopolski and Calov [38] . CO 2 , N 2 O and CH 4 are time dependent [39] , [40] , [41] . The N 2 O record is incomplete over the last 150,000 years. Given the strong resemblance with millennial CH 4 variability [41] , N 2 O values were scale to the CH 4 signal to obtain a continuous N 2 O record. The daily mean irradiance is calculated following Berger [42] . For the transient simulation, the Bering strait is closed. The effect of glacial-interglacial sea-level changes on the bathymetry and on the seawater salinity is neglected. We also realized 30 years of simulation with daily output every 5,000 years for the last 150,000 years. Identification of past summer monsoon periods requires the inclusion of shifts in the seasons with time [32] . For example, the late summer monsoon in autumn is critically depending on the definition of the season [32] . To tackle this issue, we applied here a specific strategy. Rather than choose and fix specific months for the summer monsoon, we first identified the warmest month over the Indo-Asian continent (10–35°N and 70–120°E) and the following 3 rainy months in South Asia (~17°N–33°N and 87°E–116°E). If the month before the 3 months identified is more intense in terms of precipitation, it was considered as the first month of the summer monsoon. This definition makes sense as the summer monsoon is triggered by the sensible heat difference between the ocean and the continent (that is, when continental temperatures are maximal). We then applied a criterion to account for a potential fourth month of precipitation to take into account the length of the rainy season in our definition. A fourth month of precipitation was included in our summer monsoon period if the precipitation exceeds 75% of the mean previous 3 months. Therefore, our summer monsoon period is defined independently of any specific season and its change in the past takes into account the length of the rainy season. Calcite δ 18 O computation and comparison The δ 18 O in precipitation obtained in the South Asia region (~17°N–33°N and 87°E–116°E) was corrected from the ice-sheet contribution to the global seawater δ 18 O over the last 150,000 years [43] ( Fig. 2a ). We then computed annual mean calcite δ 18 O from δ 18 O in precipitation and atmospheric temperature ( Fig. 2a,b ) using an equation for synthetic calcite under equilibrium conditions [22] . We choose the atmospheric temperature at 2 m in our model to compute annual mean calcite δ 18 O. Temperature at 2 m is not expected to faithfully reflect the cave temperature, since the diffusion of temperature from the surface to the inside of the cave is dependent on many factors such as soil structure, depth of the cave, rock environment and so on. The mean temperature in a specific cave is thus expected to be offset with respect to the mean temperature at 2 m. A weak but significant correlation ( R 2 =0.63) has been observed for the present day between cave temperature and modelled annual mean atmospheric temperature at the global scale [37] . Furthermore, the main factor in our analysis is the temperature anomaly with respect to the present day. Using temperature at 2 m is thus equivalent to assuming a constant offset between surface and cave temperature. The modelled temperature is also regionally consistent with annual reconstructed variations in south Asia between the last glacial maximum and present of ~3 °C (refs 44 , 45 ) ( Fig. 2b ). Sanbao records exhibit lower calcite δ 18 O values (by ~1.6‰) in comparison with Hulu and Dongge cave records [4] , [9] . This offset can be explained by the differences in elevations and temperatures of the cave sites. The elevation and mean temperature at the Sanbao cave are 1.800 m higher and 6–7 °C lower than at the Hulu cave [4] . The comparison between data and i LOVECLIM model results for present-day calcite δ 18 O in the Asian region is good overall ( Supplementary Fig. 10 ). However, considering (1) that the calcite δ 18 O signal exhibits differences in terms of absolute values between Hulu, Dongge and Sanbao sites [3] , [4] , [5] , [9] and (2) some difficulties to simulate the exact absolute values of speleothems with iLOVECLIM [37] at the global scale (although the amplitude of changes is correctly reproduced [44] ), all the data (Hulu, Sanbao and Dongge) and model results ( i LOVECLIM) were centred for comparison (the mean was subtracted). How to cite this article: Caley, T. et al . Orbital Asian summer monsoon dynamics revealed using an isotope-enabled global climate model. Nat. Commun. 5:5371 doi: 10.1038/ncomms6371 (2014).